Structural and functional conservation of fungal MatA and human SRY sex-determining proteins Sex determination in animals and fungi is regulated by specific sex-determining genes. The Aspergillus nidulans mating type gene matA and the human SRY (Sex-Determining Region Y) encode proteins containing a single HMG (high-mobility group) domain. Analysis of the amino-acid sequence of MatA and SRY transcription factors revealed significant structural similarity. The human SRY protein is able to functionally replace MatA and drives the sexual cycle in the fungus A. nidulans . Functional studies indicate that SRY drives early fruiting body development, and hybrid MatA protein carrying the SRY HMG box is fully capable of driving both early and late stages of sexual development, including gametogenesis. Our data suggest that SRY and MatA are both structurally and functionally related and conserved in regulating sexual processes. The fundamental mechanisms driving evolution of the genetic pathways underlying sex determination, sex chromosomes and sexual reproduction in eukaryotes appear similar. Fungal mating-type systems demonstrate remarkable structural parallels between Mat loci and sex chromosomes in mammals, which suggest similar mechanisms may have operated in divergent eukaryotes during the early evolution of sex determination and sex chromosomes. It has long been recognized that fungal Mat loci share structural and functional features with the mammalian X and Y sex determination system [1] , [2] , [3] , [4] , [5] . The classic examples involve ascomycete Neurospora tetrasperma and basidiomycete Cryptococcus neoformans, where mating type loci encode several sex-specific genes. These genes occupy large recombination-suppressed regions and similar to sex chromosomes in animals are rich in repetitive elements. The functional conservation of sex-determining genes between distantly related eukaryotes such as fungi and mammals remains unclear. In this report, we describe structural similarity and functional conservation between the MatA (high-mobility group (HMG) box) protein of ascomycete Aspergillus nidulans and human sex determination region of the Y chromosome (SRY). Sex-determining HMG-domain proteins of fungal and mammalian origin belong to the SOX/MATA/TCF superfamily of transcriptional regulators containing a single HMG domain. These proteins typically bind to the minor groove of a specific DNA sequence and act as architectural factors bending the DNA and facilitating gene transcription through changes in the chromatin structure [6] , [7] . The role of HMG domain proteins in sex determination have focused on mammalian models. We hypothesize that structural similarity between fungal MatA and human SRY reflects functional relatedness between both HMG box proteins in the process of sex determination. Structural comparisons Analysis of the amino-acid sequence of MatA (318aa) and SRY (204aa) transcription factors revealed a remarkable level of structural similarity ( Fig. 1a ), which suggests that MatA is a structural homologue of human SRY. The HMG domain region contains 33% identity and 58% positives between conserved amino acids. The SRY HMG domains from human and various mammalian species share 70% identity [8] . Interestingly, human and murine SRY/Sry factors exhibit a remarkable sequence divergence with essentially no homology outside the HMG-box [8] . Mouse Sry contains a glutamine-rich region that is completely absent in human. Sequences outside the HMG box in MatA and hSRY are less conserved, although patches of closely similar sequence can be easily identified in both N- and C-terminal protein regions. The C-terminal conservation of putative helix 3 with the His, Tyr and Pro residues suggests potential similar DNA-bending capacity. Surprisingly, there appears to be a higher level of structural conservation in the N- and C-terminal regions between fungal MatA and hSRY than between mouse Sry and human SRY. This supports the observation that mouse SRY is highly divergent based on microsatellite instability [9] . 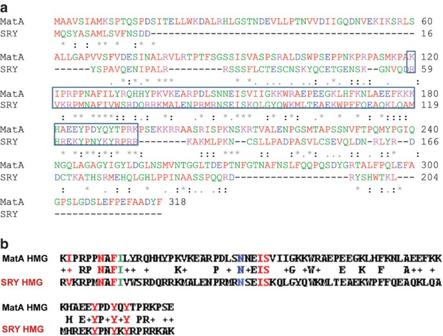Figure 1: Structural amino-acid comparison of MatA and SRY. (a) Mating type protein MatA is a structural homologue of human SRY. Pairwise alignment of the amino-acid residues in MatA and SRY. The HMG box is shaded in grey. Colour residue reflects physical-chemical nature of amino acids. Red (small, hydrophobic), blue (acidic), magenta (basic), green (hydroxyl, amine, basic). Level of conservation is indicated; (*) residue is identical, (:) conserved substitutions, (.) semi-conservative substitutions. (b) The HMG box of fungal MatA is highly similar to the HMG box of human SRY. Pairwise sequence alignment of the HMG box from MatA and SRY HMG. Conserved and similar (+) residues are indicated in the centre line. All residues marked in colour represent key amino acids making direct contact with DNA. Amino acids marked in red are involved in binding to the specific DNA core sequence. Isoleucine (I) marked in green is involved in binding the minor groove of DNA. Asparagine (N) marked in blue is typical of HMG boxes binding DNA in a sequence-specific manner. Figure 1: Structural amino-acid comparison of MatA and SRY. ( a ) Mating type protein MatA is a structural homologue of human SRY. Pairwise alignment of the amino-acid residues in MatA and SRY. The HMG box is shaded in grey. Colour residue reflects physical-chemical nature of amino acids. Red (small, hydrophobic), blue (acidic), magenta (basic), green (hydroxyl, amine, basic). Level of conservation is indicated; (*) residue is identical, (:) conserved substitutions, (.) semi-conservative substitutions. ( b ) The HMG box of fungal MatA is highly similar to the HMG box of human SRY. Pairwise sequence alignment of the HMG box from MatA and SRY HMG. Conserved and similar (+) residues are indicated in the centre line. All residues marked in colour represent key amino acids making direct contact with DNA. Amino acids marked in red are involved in binding to the specific DNA core sequence. Isoleucine (I) marked in green is involved in binding the minor groove of DNA. Asparagine (N) marked in blue is typical of HMG boxes binding DNA in a sequence-specific manner. Full size image Comparison of the HMG box of fungal MatA and human SRY reveals unexpectedly high conservation of the amino-acid sequence ( Fig. 1b ). All ten amino-acid residues that are known to form a direct contact with the DNA helix [10] are identical between fungal and human HMG boxes. Residues marked in red are known to participate in a sequence-specific binding of HMG domain to the core DNA sequence [10] . As shown, all residues marked in red are identical except for the isoleucine (I) in MatA and valine (V) in SRY at position 2, which are non-identical but have similar physico-chemical properties. The asparagine (N), highlighted in blue, is typical of HMG boxes binding to DNA in a sequence-specific manner [11] , and as indicated these residues are identical. Furthermore, the isoleucine (I) highlighted in green is important for HMG box-specific DNA-bending and -binding efficiency [8] , [12] , [13] . The conservation of isoleucine residue in both fungal and human HMG boxes may reflect similar modes of DNA binding and bending. MatA also contains a cluster of basic residues (ASRISPKN), which is similar to a cluster (KAKMLPKN) found in the SRY-related proteins. These residues are located C-terminal to the HMG box and are known to function as a kinetic clamp to prolong the lifetime of SRY–DNA complex [14] . These conserved residues also provide insights into the ancestral origins of SRY compared with MatA, which are thought to be duplication events (for example, SOX3, TCF-1 and LEF-1) that can impact nucleocytoplasmic trafficking [15] . Functional comparison The structural similarity between fungal MatA and human SRY may suggest a functional conservation in the sex-determining pathway or other pathways driving sexual reproduction. To further explore this possibility, we used the fungal model A.nidulans to perform interspecies gene exchange studies and analyse the ability of the human SRY protein to drive fungal sexual cycle. Manipulations of the matA gene structure and associated phenotypes of the resulting transgenic fungal strains are outlined in Fig. 2 . The endogenous open reading frame (ORF) of the matA gene was replaced with the ORF sequence of the SRY, creating a transgenic A. nidulans strain carrying the SRY ORF under control of the matA promoter. A separate transgenic strain was created, where the matA promoter: SRY transgene was integrated ectopically into the genome of a matA(0) strain lacking endogenous matA . Therefore, two independent strains were created (for example, endogenous and ectopic) and tested with consistent phenotypes found, although the ectopic transgene was less robust. In addition, Southern blot, PCR and DNA-sequencing methods were all used to validate the different strains for SRY and SRY-MatA hybrid strains, see Methods [16] and Supplementary Fig. 1 . The matA(0) strains have a sterile phenotype described previously [16] . Sexual development of the ORF swap strains was analysed with reference to the wild-type matA -positive control strain and matA(0) deletion-negative control strain. At the early stage of the sexual cycle, 4–5 days post induction, the wild-type strain differentiated abundant fruiting bodies (cleistothecia; Fig. 3 -1C). By contrast, matA (0) and ORF swap strains lacked fruiting bodies and had developed only clusters of white hülle cells, which is typically an indication of unsuccessful fertilization ( Fig. 3 -4C). However, at 2 weeks post induction, the wild-type strain had developed mature cleistothecia (100–200 μm in diameter) with abundant meiotic progeny (ascospores; Fig. 3 -1A,B,C). The matA(0) strain showed no progress in further sexual development, forming thick masses of hülle cells with occasional formation of tiny, undeveloped progenitors of cleistothecia and no ascospores ( Fig. 3 -4A,B,C). The ORF swap strain at the corresponding time point differentiated small (50–100 μm) cleistothecia at approximately 20–30% of the wild-type fruiting body abundance ( Fig. 3 -3B). These cleistothecia were mostly barren with development of the internal reproductive tissue having been aborted at the early stage of ascogenous hyphae differentiation. However, a small number of viable ascospores were observed ( Fig. 3 -3A,B,C). Ascospore viability was routinely assessed by plating spores on agar plates, incubating and counting growing colonies. Viability of ascospores isolated from ORF swap strains and sexual phenotypes were stable generationally and meiotically that resolves secondary mutation effects. Therefore, human SRY is able to partially support fungal sexual differentiation, although formation of the meiotic progeny is inefficient. Partial function of the SRY protein in driving fungal sexual development could be a result of impaired DNA binding and/or bending because of the lack of sufficient conservation between the MatA and SRY proteins. Other possibilities may include failures in protein–protein interactions between SRY and MatA-interacting fungal proteins, altered posttranslational modifications, or improper recognition of the downstream sex-specific target genes. Limited information is currently available regarding downstream gene targets for MatA, but future studies may help elucidate if altered gene expression may be a factor. Any of these abnormalities could contribute to the partial function of SRY in regulating fungal sexual development. 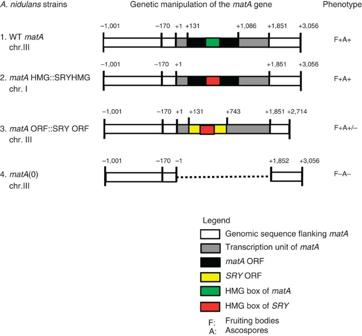Figure 2: Genetic manipulations of thematAlocus. Schematic outline illustrating structure ofmatAin wild-typeA.nidulansand its derivative strains carrying the ORF or HMG box of SRY. The genomic, chromosomal (chr.) location of the ectopic fusion gene is indicated. (1) Structure of WTmatAgene. (2) The HMG box ofmatAreplaced with HMG box of SRY. (3) The ORF ofmatAreplaced with the ORF of SRY. (4) Mutant carrying complete deletion ofmatA. Associated sexual cycle phenotypes are summarized. The elements of gene structure are distinguished by different colour (legend), the distance in base pairs (bp) is shown. Figure 2: Genetic manipulations of the matA locus. Schematic outline illustrating structure of matA in wild-type A.nidulans and its derivative strains carrying the ORF or HMG box of SRY. The genomic, chromosomal (chr.) location of the ectopic fusion gene is indicated. (1) Structure of WT matA gene. (2) The HMG box of matA replaced with HMG box of SRY. (3) The ORF of matA replaced with the ORF of SRY. (4) Mutant carrying complete deletion of matA . Associated sexual cycle phenotypes are summarized. The elements of gene structure are distinguished by different colour (legend), the distance in base pairs (bp) is shown. 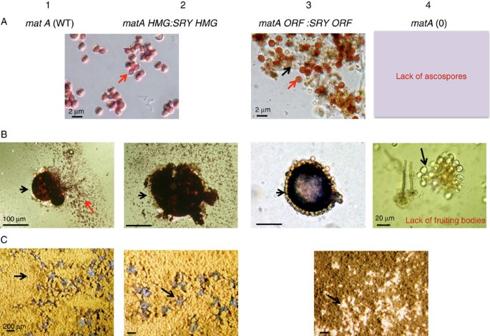Figure 3: Human HMG box of SRY drives sexual cycle inA. nidulans. Column 1: Sexual differentiation in wild-typeA.nidulans. Mature ascospores (red arrow), Column 1-A. Individual, crushed fruiting body (black arrow) with released ascospores (red arrow), Column 1-B. Abundant, spherical fruiting bodies (purple-black balls) develop within the vegetative tissue among yellow conidiating conidiophores (black arrow), Column1-C. Column 2: The HMG box of SRY supports a wild-type sexual cycle. Abundant fruiting bodies, Column 2-B,C. Representative image of wild-type mature ascospores is shown for both WT and HMG box swap strains in Columns 1-A/2-A. Column 3: The SRY ORF partially restores sexual cycle. Scarce fruiting bodies form within clusters of hülle cells, Column 3-B,C. Ascogenous tissue is mostly undeveloped, Column 3-A (black arrow), with small number of mature and viable ascospores, Column 3-A (red arrow). Column 4: ThematA (0)complete knockout is sterile, does not produce fruiting bodies or ascospores, Column 4-A, only clusters of hülle cells are formed, Column 4-B,C (arrows). Full size image Figure 3: Human HMG box of SRY drives sexual cycle in A. nidulans . Column 1: Sexual differentiation in wild-type A.nidulans . Mature ascospores (red arrow), Column 1-A. Individual, crushed fruiting body (black arrow) with released ascospores (red arrow), Column 1-B. Abundant, spherical fruiting bodies (purple-black balls) develop within the vegetative tissue among yellow conidiating conidiophores (black arrow), Column1-C. Column 2: The HMG box of SRY supports a wild-type sexual cycle. Abundant fruiting bodies, Column 2-B,C. Representative image of wild-type mature ascospores is shown for both WT and HMG box swap strains in Columns 1-A/2-A. Column 3: The SRY ORF partially restores sexual cycle. Scarce fruiting bodies form within clusters of hülle cells, Column 3-B,C. Ascogenous tissue is mostly undeveloped, Column 3-A (black arrow), with small number of mature and viable ascospores, Column 3-A (red arrow). Column 4: The matA (0) complete knockout is sterile, does not produce fruiting bodies or ascospores, Column 4-A, only clusters of hülle cells are formed, Column 4-B,C (arrows). Full size image HMG box comparison Structural and functional analyses of the mammalian HMG box proteins suggest that the conserved DNA-binding HMG motif is necessary and sufficient element of SRY protein required to initiate male development and sex determination [17] . Indeed, most point mutations causing human sex reversal occur de novo in the HMG box region and impair specific DNA binding or DNA bending affecting the assembly of sex-specific transcriptional complexes [8] , [14] . Several studies in mice demonstrated that transgenic expression of mammalian SRY or SOX protein bearing an SRY-type HMG domain within the mouse embryonic gonad during the critical time frame was sufficient to trigger male sex determination and XX sex reversal [17] , [18] . Exploring this idea further we sought to investigate whether the SRY HMG box can functionally replace the MatA HMG box and be sufficient to regulate the A.nidulans sexual cycle. The HMG box of MatA was replaced with the HMG box of SRY and a transgene carrying the HMG swap was integrated ectopically into the matA(0) genome. Several independently derived HMG box swap transformants were analysed and showed consistent phenotypes. We found that the hybrid MatA protein containing an HMG box of SRY is able to support a robust sexual cycle with fruiting body and progeny formation ( Fig. 3 -2A,B,C). These data reveal functional conservation of the human HMG box within the context of fungal MatA protein in driving fungal sexual reproduction. Regulatory element comparison Interestingly, the structural conservation between MatA and SRY extends outside the gene-coding region. Analysis of the promoter region in matA and SRY genes reveals a number of conserved putative regulatory elements. The promoter region of the mammalian SRY has several potential binding sites for SRY protein [19] . The HMG domain-specific core sequences (AACAAAG) have been identified 94 bp upstream of the ATG in human SRY [20] , and in several other mammalian species [19] . Analogously, we identified an identical sequence (CAAAG) located 216 bp upstream of the translational start codon ATG of matA gene in A. nidulans . Furthermore, we identified a sequence for a potential silencing element residing in the 5' matA flank (−931 to −960 bp), which shares high similarity to the putative silencing element found in the upstream regulatory region of the SRY gene ( Fig. 4 ) [19] . Although this region has a number of regulatory elements nearby that are similar for a number of different species, deletion of this region in studies for the Wilms’ Tumour 1 (WT1), Gata4 or TFCP2 did not show strong regulatory activity in SRY reporter gene analysis [21] , [22] , [23] . Similarly, deletion of this element does not affect matA expression in vivo or sexual development [16] . Interestingly, we identified a functional silencer, matA SE, located between −512 and −248 bp that bears limited similarity to hSRY SE [16] ( Fig. 4 ). This general region also has a large number of regulatory elements (for example, WT1, Gata4, Cp2) that are functional in SRY [19] , [21] , [22] , [23] , [24] . The structural conservation of these regulatory elements suggests similar mechanisms might be involved in the transcriptional regulation and expression of matA and SRY ( Fig. 4 and Supplementary Fig. 2 ). These elements [24] in both matA [16] and SRY [19] appear to have been evolutionarily conserved and may contribute to the regulation of gene expression [16] , [19] , [24] . 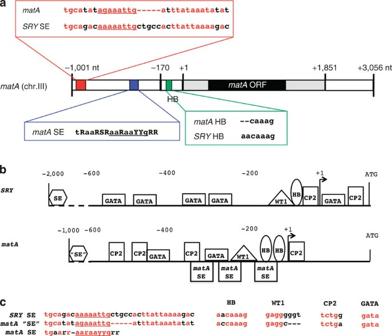Figure 4: Structural conservation of the promoter regions inSRYandmatAgenes. (a) The putative HMG-binding sequence (HB), sequence element similar tohSRYSE and functionalmatASE have been identified in the proximal and distal region ofmatApromoter. (b) Schematic representation showing the distribution and location of binding sites for transcription factors. Binding sites recognized by WT1, Gata4 and Cp2 are indicated. Hexagonal shape (silencing element, SE/‘SE’) indicates position of conserved but apparently non-functional sequence related to MHC1 silencer. Square shape (matA SE) indicates positions of the functional silencer elements inA.nidulans. Oval shape (HMG-box binding, HB) indicates sites for putative binding of SRY and MatA proteins. Arrows indicate transcriptional start sites. (c) Alignment of the consensus DNA sequence for the putative regulatory elements identified in the promoter regions ofSRYandmatA. Level of homology and conservation is showed. Underlined bases within the silencer regions indicate binding sites for the silencer of MHC class I gene. Figure 4: Structural conservation of the promoter regions in SRY and matA genes. ( a ) The putative HMG-binding sequence (HB), sequence element similar to hSRY SE and functional matA SE have been identified in the proximal and distal region of matA promoter. ( b ) Schematic representation showing the distribution and location of binding sites for transcription factors. Binding sites recognized by WT1, Gata4 and Cp2 are indicated. Hexagonal shape (silencing element, SE/‘SE’) indicates position of conserved but apparently non-functional sequence related to MHC1 silencer. Square shape (matA SE) indicates positions of the functional silencer elements in A.nidulans . Oval shape (HMG-box binding, HB) indicates sites for putative binding of SRY and MatA proteins. Arrows indicate transcriptional start sites. ( c ) Alignment of the consensus DNA sequence for the putative regulatory elements identified in the promoter regions of SRY and matA . Level of homology and conservation is showed. Underlined bases within the silencer regions indicate binding sites for the silencer of MHC class I gene. Full size image Chromosomal sex-determining regions have evolved independently in different eukaryotic species and undergone a convergence of structure and function [1] , [2] , [3] . Consistent with this theory, it has been speculated that fungal Mat idiomorphs may represent primitive forms of sex chromosomes [1] , [2] , [25] , [26] . The current observations highlight a remarkable structural similarity and functional conservation between the fungal MatA and human SRY sex-determining factors. The HMG box of human SRY is able to functionally replace the HMG box of fungal MatA and drives robust sexual differentiation and gametogenesis in A. nidulans. Combined observations provide insights concerning the role and conservation of the HMG box proteins in regulation of genetic pathways underlying sex determination and sexual reproduction in eukaryotes. Clearly, other transcription factors such as homeodomain proteins for fungi and mammals are required [27] , [28] . For example, previous analysis of DM domain proteins, such as DMRT or DMY, have strong conservation across metazoan sexual development, from insects to mammals [25] . Therefore, different classes (for example, HMG and DM) of transcription factors known to be involved in sex determination are also likely to have similarities between the mammalian and fungal processes. The current study suggests HMG domain proteins such as MatA and SRY have a strong conservation in sexual development, from fungi to mammals. Therefore, a combination of HMG box proteins, and potentially other factors such as DM domain proteins, appear to be involved in the sexual development of most organisms. Protein sequence analysis Amino-acid sequences of the MatA (AN4734.3) and SRY (Q05066) proteins were analysed using Clustal W multiple sequence alignment using the European Bioinformatics Institute website services at http://www.ebi.ac.uk/Tools/clustalw2/index.html . Vectors construction The SRY-coding region (612 bp) was amplified from the human genomic DNA using primers SRYF1 (5′-ATGCAATCATATGCTTCTGCTATG-3′) and SRYR1 (5′-CTACAGCTTTGTCCAGTGGCT-3′). The SRY fragment was cloned into the Topo cloning pcr8 vector (pcr8-SRY). The ORF swap destination vector pmat:SRYORF:mat containing the SRY ORF under regulation of the matA promoter and terminator was created as a result of recombination reaction between the pcr8-SRY and pmatAORF swap vector [29] . The human SRY HMG box was amplified using the primers hSRYF2 (5′-AGAGTGAACCGACCCATGAAC-3′) and hSRYR2 (5′-CCGACGAGGTCGATACTTATAATTC-3′). The An matA sequence 5′ of the HMG box was amplified by using AnmatAF10 (5′-AGTGAGGGTAGAGTCTAC-3′) and AnmatHMGswapR (5′-P i TGCGGGTTTCATTGACGCTGGC-3′). The An matA sequence downstream of the HMG box was amplified using AnmatHMGswapF (5′-P i CCTTCTGAAAAGAAGCGTCGTG-3′) and AnmatAR10 (5′-TGGAACTCCAGGAGCCGCTCGA-3′). The three products were then ligated and the resultant ligation product amplified using AnmatAF26 (5′-GGACGAAAAGCTTCTGCATTC-3′) and AnmatAR11 (5′-TGCCGTATGCTACCTGAGC-3′). The PCR product that corresponded to the predicted size of the chimeric gene was then topo cloned into pcr8. The resultant clone was purified and validated with DNA sequencing. The matA/SRY HMG box fusion gene was transferred into an An pyrG vector (pAn7) using the Invitrogen clonase system to create pmatHMGswap. Transformation and targeted gene replacement in A. nidulans Two independent ORF swap and multiple HMG box swap strains have been created. A. nidulans UI461 ( yA 2, pabaA 1, pyroA 4, argB 2, matA (0):: AfargB , nku :: bar ) and UI 465 ( yA 2, pyrG 89, pabaA 1, matA (0):: AfargB, nku::bar ) were used as the recipient strains. Plasmids: pmatAORF:SRYORF and ppyro were co-transformed into the UI461 strain. About 200 individual transformants that stably integrated the ppyro plasmid were recovered. All transformants were subsequently screened on YGMTV media for a non-conidiating phenotype indicative of arginine auxotrophy. Loss of arginine prototrophy indicates homologous recombination and a gene replacement event where the mat:SRYORF:mat fusion construct replaced the endogenous matA (0):: AfargB . Out of 200 transformants, 1 argB - colony was isolated, transformant T52. Gene replacement and correct integration of matAORF: SRYORF construct was confirmed by Southern blot, PCR and DNA-sequencing analysis ( Supplementary Fig. 1 ). Arginine auxotrophy impairs sexual reproduction, therefore the transformant T52 was subsequently transformed with the pargB plasmid to confer arginine prototrophy. Several, independent single ascospore isolates were also derived from viable ascopspores produced by the original T52 argB + strain. The ORF swap construct was also integrated ectopically into the UI465 strain carrying matA (0) at the resident location. Vector pmatHMGswap was used to create the HMG box swap strain by transforming UI465 strain. Routinely with all stains Southern blots, PCR and DNA sequencing were performed to identify and validate the transformants with a single copy of the plasmid integrated at pyrG. Multiple independent strains on different genetic backgrounds were determined for all constructs and tested. Analysis of the sexual phenotype Sexual development of wild-type matA (A1153), matA (0)UI461and mat:hSRY:mat (UI470) was induced under standard culture condition as previously described [16] , [29] . Development of hülle cells, protocleistothecia and cleistothecia were monitored over a 2-week period. Viability of ascospore fruiting bodies were routinely measured by plating spores on agar plates, incubating and counting growing colonies. How to cite this article: Czaja, W. et al. Structural and functional conservation of fungal MatA and human SRY sex-determining proteins. Nat. Commun. 5:5434 doi: 10.1038/ncomms6434 (2014).